Structure of dual receptor binding to botulinum neurotoxin B Botulinum neurotoxins are highly toxic, and bind two receptors to achieve their high affinity and specificity for neurons. Here we present the first structure of a botulinum neurotoxin bound to both its receptors. We determine the 2.3-Å structure of a ternary complex of botulinum neurotoxin type B bound to both its protein receptor synaptotagmin II and its ganglioside receptor GD1a. We show that there is no direct contact between the two receptors, and that the binding affinity towards synaptotagmin II is not influenced by the presence of GD1a. The interactions of botulinum neurotoxin type B with the sialic acid 5 moiety of GD1a are important for the ganglioside selectivity. The structure demonstrates that the protein receptor and the ganglioside receptor occupy nearby but separate binding sites, thus providing two independent anchoring points. Botulinum neurotoxins (BoNT) are the most toxic substances known, with a lethal dose (LD 50 ) value of ~1 ng kg −1 (ref. 1 ). Seven distinct serotypes of BoNTs (A-G) exist [2] , [3] . Because of their extreme toxicity, they are one of the top potential bioterrorism agents. However, members of the BoNTs (BoNT/A and B) are also extensively used therapeutically to treat numerous medical conditions, such as cervical dystonia, cerebral palsy, strabismus, hemifacial spasm and myofascial pain, as well as for cosmetic purposes [4] , [5] , [6] . These toxins are composed of three domains: the light chain (LC), the translocation domain (H N ) and the binding domain (H C ). The LC (~50 kDa), is a Zn-protease responsible for the cleavage of the SNARE (soluble NSF attachment protein receptor) proteins targeted by the toxin. SNARE proteins are central in synaptic vesicle exocytosis; cleavage of SNARE proteins by BoNTs inhibits acetylcholine release at the neuromuscular junctions [7] . H N (~50 kDa) is responsible for transport of the LC over the endosomal membrane. H C (~50 kDa) binds to receptors on nerve terminals [2] , [8] , [9] . H C is further divided into H CN and H CC , with H CN being highly conserved and H CC being diverse in sequence. The receptors bound by H CC and the final protein being targeted by the LC varies between serotypes. In general, BoNTs achieve their high affinity and specificity for neurons by binding two receptors; gangliosides and one of the two synaptic vesicle proteins, synaptotagmin (Syt) or synaptic vesicle protein 2 (SV2). BoNT/A, D and E use SV2 as their protein receptor [10] , [11] , [12] , [13] , BoNT/F might also utilize SV2 [14] , [15] , although this has not been functionally confirmed [13] , [16] . BoNT/B and BoNT/G as well as a BoNT subtype, type DC, bind Syt, both the Syt-I and Syt-II isoforms, as their protein receptors [17] , [18] , [19] , [20] , [21] , [22] , [23] , [24] . Gangliosides bind in a ganglioside-binding site (GBS), conserved in all serotypes except C and D, consisting of a SXWY motif [14] , [15] , [25] , [26] , [27] , [28] , [29] , [30] . BoNT/C and D have in the same site an analogous GBS [31] , [32] , [33] . Independent of which receptor the BoNT bind, the end result is similar; cleavage of SNARE proteins by the LC leading to muscle paralysis [8] . Structures showing BoNT binding to either its protein receptor or gangliosides alone have been reported, including BoNT/B in complex with its protein receptor, synaptotagmin II (Syt-II) [19] , [22] , BoNT/A with ganglioside GT1b [28] and BoNT/F with ganglioside GD1a [34] . Structures are also available for BoNT/B, C and D bound to smaller sugars [25] , [31] , [33] , [35] . However, how BoNTs bind to both protein receptors and gangliosides simultaneously remains to be established at the structural level. Furthermore, no structure of BoNT/B bound to a complex ganglioside has previously been determined. Here, we solve the structure of the first ternary complex of a BoNT bound to both its protein receptor and ganglioside. We determine the 2.3-Å structure of BoNT/B bound to Syt-II and the ganglioside GD1a. We show that the binding of GD1a does not influence the toxins affinity for Syt-II. Our results show that the two receptor-binding sites are independent of each other. Overall structure of the complex In a similar approach as previously reported, BoNT/B-H C was constructed and purified as a fusion construct together with Syt-II [22] . This recombinant protein was then pre-incubated with GD1a, a major brain ganglioside known to bind BoNT/B [36] , devoid of the ceramide part. 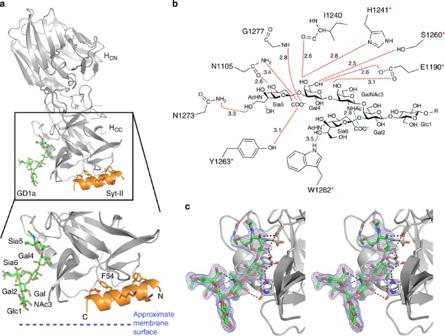Figure 1: Dual receptor binding to BoNT/B. (a) Overall view of BoNT/B (grey) with GD1a (green) and mouse Syt-II (orange) bound. Lower panel shows a close-up view on the GD1a- and Syt-II-binding sites, with the GD1a moieties and the Syt-II residues, interacting with BoNT/B, shown as sticks. Phenylalanine 54 is indicated, this position is a leucine in human Syt-II that has a drastically lower affinity to BoNT/B than mouse Syt-II17,44. (b) Schematic overview of possible hydrogen bonds between GD1a and BoNT/B (red dashed lines) and an internal hydrogen bond (blue dashed line). The hydrogen bond distance is shown for each bond (Å). Red stars show residues that previously, via mutagenesis, have been shown to be important for ganglioside binding26. In GD1a, a ceramide is present at the R position, the GD1a oligosaccharide used here has a hydrogen in this position. (c) Stereo view of the bound GD1a, with its electron density (2 FO-FCmap contoured at 1.5σ) in blue, and the possible hydrogen bonds to BoNT/B residues as dashed lines. Subsequent co-crystallization experiments yielded crystals that diffracted to 2.3 Å ( Table 1 ). The structure was solved using molecular replacement. Residues 862–1291 of BoNT/B-H C were visible in the electron density, with the exception of two flexible loops between residues 1,151–1,159 and 1,245–1,252. Well-defined electron density became visible during refinement, accounting for both the fused Syt-II toxin-binding region (residues 45–59), and the entire GD1a ganglioside sugar ( Fig. 1a ). The remainder of the fused Syt-II was disordered and not visible in the electron density. The asymmetric unit contained two BoNT/B molecules, which were virtually identical (root-mean squared deviation of 0.4 Å). Table 1 Data collection and refinement statistics Full size table Figure 1: Dual receptor binding to BoNT/B. ( a ) Overall view of BoNT/B (grey) with GD1a (green) and mouse Syt-II (orange) bound. Lower panel shows a close-up view on the GD1a- and Syt-II-binding sites, with the GD1a moieties and the Syt-II residues, interacting with BoNT/B, shown as sticks. Phenylalanine 54 is indicated, this position is a leucine in human Syt-II that has a drastically lower affinity to BoNT/B than mouse Syt-II [17] , [44] . ( b ) Schematic overview of possible hydrogen bonds between GD1a and BoNT/B (red dashed lines) and an internal hydrogen bond (blue dashed line). The hydrogen bond distance is shown for each bond (Å). Red stars show residues that previously, via mutagenesis, have been shown to be important for ganglioside binding [26] . In GD1a, a ceramide is present at the R position, the GD1a oligosaccharide used here has a hydrogen in this position. ( c ) Stereo view of the bound GD1a, with its electron density (2 F O -F C map contoured at 1.5 σ ) in blue, and the possible hydrogen bonds to BoNT/B residues as dashed lines. Full size image The structure shows that Syt-II is bound in a hydrophobic crevice on the tip of BoNT/B ( Fig. 1a ). The overall structure obtained in the ternary complex is virtually identical to the previously reported BoNT/B·Syt-II complex structures [19] , [22] , demonstrating that simultaneous ganglioside binding does not cause any significant structure changes in BoNT/B. Ganglioside binding to BoNT/B This is the first structure of BoNT/B in complex with a complex ganglioside. The GBS on BoNT/B has been previously mapped, mainly through mutagenesis studies, and contains a conserved SXWY motif [26] . The ternary complex structure revealed that GD1a indeed binds to this established GBS ( Figs 1 and 2 ). Four subunits of GD1a (sialic acid (Sia5), galactose (Gal4), N -acetylglucosamine (GalNAc3) and Sia6) make contacts to the GBS of BoNT/B ( Fig. 1b ). Sia5 forms hydrogen bonds to N1273, N1105, G1277 and Y1263, Gal4 to I1240, H1241, S1260 and E1190. GalNAc3 and Sia6 form one hydrogen bond each, to E1190 and W1262, respectively. W1262 is furthermore forming crucial aromatic stacking interactions with Gal4. The remaining two subunits of GD1a, Glc1 and Gal2, do not interact with the GBS, but are still visible in the electron density due to the crystal packing to the second monomer in the asymmetric unit ( Fig. 3 ). These crystal contacts are not biologically relevant; BoNT/B has previously been shown to have a single GBS [26] . Key residues in the GBS mapped by previous mutagenesis studies, are highlighted with a star in the figure ( Fig. 1b ) [26] . 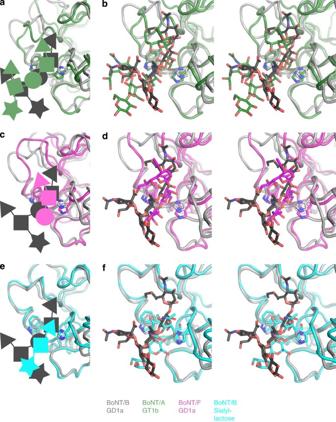Figure 2: Comparison of the ganglioside binding to BoNT/B, BoNT/A and BoNT/F. The residues corresponding to W1262 and H1241 are shown in all structures. In the schematic panels (a,c,e) the individual sugar moieties are depicted as follows; triangles, Sia; rectangles, Gal; circle, GalNAc; star, Glc. In all panels, BoNT/B with GD1a bound is depicted in grey and dark grey, respectively. The right-hand panels (b,d,f) are stereo figures of the GBS. (a,b) Comparison to BoNT/A with GT1b (green, PDB code:2VU9). (c,d) Comparison to BoNT/F and its bound GD1a (magenta, PDB code:3RSJ). (e,f) Comparison to BoNT/B and its bound sialyllactose (cyan, PDB code:1F31). Figure 2: Comparison of the ganglioside binding to BoNT/B, BoNT/A and BoNT/F. The residues corresponding to W1262 and H1241 are shown in all structures. In the schematic panels ( a , c , e ) the individual sugar moieties are depicted as follows; triangles, Sia; rectangles, Gal; circle, GalNAc; star, Glc. In all panels, BoNT/B with GD1a bound is depicted in grey and dark grey, respectively. The right-hand panels ( b , d , f ) are stereo figures of the GBS. ( a , b ) Comparison to BoNT/A with GT1b (green, PDB code: 2VU9 ). ( c , d ) Comparison to BoNT/F and its bound GD1a (magenta, PDB code: 3RSJ ). ( e , f ) Comparison to BoNT/B and its bound sialyllactose (cyan, PDB code: 1F31 ). 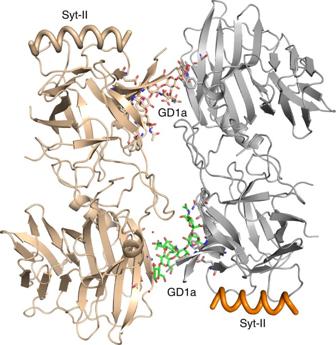Figure 3: The asymmetric unit. The asymmetric unit containing two molecules of BoNT/B (grey), with the bound recognition domain of Syt-II (orange) and GD1a (green). The second copy of each molecule is coloured in beige. All residues that interact with GD1a are shown as sticks. Crystal contacts are formed between the two BoNT/B protomers (grey and beige) in the asymmetric unit via the bound GD1a molecules. GD1a is bound to the GBS, as described inFig. 1. The crystal contacts are formed by Glc1, Gal2 and Sia6. The green GD1a forms three hydrogen bonds, to S984, N1025 and L1022. The beige GD1a forms five hydrogen bonds to S984, F986, N1025 and T1026. These interactions are not biologically relevant, as BoNT/B has been shown to have a single GBS26. Full size image Figure 3: The asymmetric unit. The asymmetric unit containing two molecules of BoNT/B (grey), with the bound recognition domain of Syt-II (orange) and GD1a (green). The second copy of each molecule is coloured in beige. All residues that interact with GD1a are shown as sticks. Crystal contacts are formed between the two BoNT/B protomers (grey and beige) in the asymmetric unit via the bound GD1a molecules. GD1a is bound to the GBS, as described in Fig. 1 . The crystal contacts are formed by Glc1, Gal2 and Sia6. The green GD1a forms three hydrogen bonds, to S984, N1025 and L1022. The beige GD1a forms five hydrogen bonds to S984, F986, N1025 and T1026. These interactions are not biologically relevant, as BoNT/B has been shown to have a single GBS [26] . Full size image We next compared the structure of BoNT/B·GD1a with the previously reported structures of BoNT/A·GT1b [28] and BoNT/F·GD1a [34] ( Fig. 2 ). We found that there are significant differences in the position of most sugar moieties ( Fig. 2a–d ). However, the position of Gal4 is fairly conserved in all three structures. Interestingly, GD1a has shifted one unit when compared with the previously determined structure of BoNT/B with bound sialyllactose [25] ( Fig. 2e ). This shift could indicate plasticity in the binding site, with different sugars being able to occupy the binding sites in different binding registers. Alternatively, the use of a partial mimic of the ganglioside or soaking could have influenced the position [25] . BoNT/B ternary complex Importantly, the structure of BoNT/B in the ternary complex, does not undergo any significant conformational changes as compared with apo BoNT/B and the BoNT/B·Syt-II complex [19] , [22] , [25] with an H CC root-mean squared deviation of 0.4 and 0.3 Å, respectively. Binding of the receptors induces only minor adjustments of the positions of side chains in the binding sites. For instance, W1262 moves slightly in the direction of Gal4. Gal2 and Glc1 are located between the membrane and the toxin, and are likely flexible. However, even allowing these moieties to be flexible, sterical and distance restraints likely prevents the ganglioside to reach the protein receptor in BoNT/B for a direct interaction. The closest distance between GD1a and Syt-II is 15 Å. E1190 interacts with GD1a and E1191 interacts with Syt-II, this is the closest connection between the binding sites. This result further establishes that the high binding affinity mainly is the product of two independent anchoring points, with no direct interactions between the binding sites or the receptors ( Figs 1 and 4 ). Furthermore, the toxins binding to the receptors impose sterical restrains on the interaction with the membrane ( Fig. 4 ). 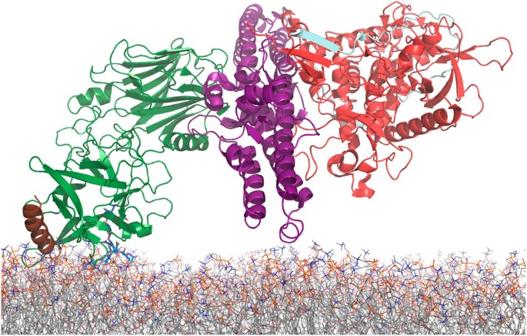Figure 4: Model of BoNT binding to the neuronal membrane. The HC(green), with its bound Syt-II (brown) and GD1a (blue), is from this study, while the HN(purple) and LC (red) is superimposed using the structure of the entire BoNT/B (PDB code:2NP0). The protein orientation is restricted by the binding of the two receptors. The structure presented here supports the entry of the translocation domain into the membrane with the end of the long helixes first22,28. The regions linking both the protein receptor and ganglioside receptor to the membrane does allow for a certain degree of flexibility of the toxins orientation. Figure 4: Model of BoNT binding to the neuronal membrane. The H C (green), with its bound Syt-II (brown) and GD1a (blue), is from this study, while the H N (purple) and LC (red) is superimposed using the structure of the entire BoNT/B (PDB code: 2NP0 ). The protein orientation is restricted by the binding of the two receptors. The structure presented here supports the entry of the translocation domain into the membrane with the end of the long helixes first [22] , [28] . The regions linking both the protein receptor and ganglioside receptor to the membrane does allow for a certain degree of flexibility of the toxins orientation. Full size image GD1a does not influence the affinity for Syt-II To further confirm the lack of allosteric effects between the dual receptors, we measured the binding affinity of rat Syt-II peptide (residues 40–60) to BoNT/B-H C , without and with a pre-incubation with GD1a oligosaccharide. Isothermal titration calorimetry (ITC) gave a K D of 0.14±0.05 μM and 0.18±0.06 μM, respectively ( Fig. 5 ). The presence of GD1a did thus not significantly affect the binding affinity between Syt-II and BoNT/B, further indicating that there is no allosteric contribution in the binding of Syt-II and GD1a. 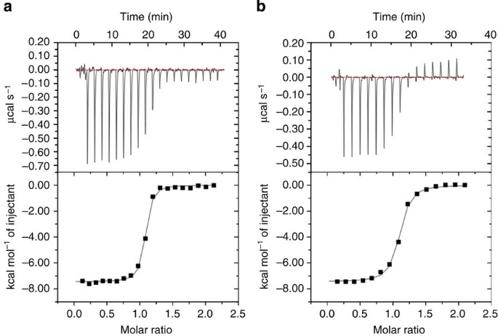Figure 5: ITC titrations of Syt-II to BoNT/B. Representative ITC titrations of Syt-II to BoNT/B, without (a) and with (b) pre-incubation of 75 μM GD1a. (a)KD=0.14±0.05 μM, (b)KD=0.18±0.06 μM. The error is the s.d. on at least two independent measurements. The baseline above zero inbis due to a slight buffer mismatch, and does not influence the calculated values. Figure 5: ITC titrations of Syt-II to BoNT/B. Representative ITC titrations of Syt-II to BoNT/B, without ( a ) and with ( b ) pre-incubation of 75 μM GD1a. ( a ) K D =0.14±0.05 μM, ( b ) K D =0.18±0.06 μM. The error is the s.d. on at least two independent measurements. The baseline above zero in b is due to a slight buffer mismatch, and does not influence the calculated values. Full size image The dual receptor concept for BoNT family toxins was proposed 27 years ago [37] . The ternary structure, of BoNT/B bound to both Syt-II and GD1a concurrently, presented here, now proves the dual receptor model at the structural level. The structure demonstrates that the binding sites are separate and there are only minor changes in the structure upon binding of the receptors. There is no allosteric contribution in the binding of Syt-II and GD1a to BoNT/B. Due to the high sequence similarity between the recognition domains of Syt-I and Syt-II, it is likely that these receptors bind the toxin in a very similar way. This is the first structure reported of BoNT/B bound to a complex ganglioside. Previous experiments have shown that GT1b and GD1a support BoNT/B binding, but that GD1b and GM1 bind substantially weaker [21] , [36] , [38] . The structure presented here reveals the structural basis for this selectivity that arises from the interactions of Sia5. The Sia5 moiety is strongly bound to BoNT/B with key interactions for the overall binding of the ganglioside. Both GT1b and GD1a have a Sia5 moiety, whereas GD1b and GM1 do not, explaining the differences in affinity. Furthermore, K1265 and R1269, close to W1262, are well positioned to interact with the second sialic acid moiety present in GT1b (but not in GD1a), likely contributing to GT1b having even higher affinity than GD1a for binding BoNT/B [25] , [36] . The detailed description of dual receptor binding to BoNT/B can be used to develop toxin countermeasures targeting both sites simultaneously, thus benefitting from the high affinity achieved by binding multiple sites, as naturally occurring in the BoNTs. Constructs and peptides The cDNA encoding BoNT/B-H C (residues 857–1291, GenBank: AB232927) was synthesized by GeneArt (Regensburg, Germany), with codon optimized for Escherichia coli expression. The cDNA encoding mouse Syt-II was generously provided by M. Fukuda (Ibaraki, Japan). The BoNT/B-H C ·Syt-II fusion construct was built by fusing BoNT/B-H C directly to the N-terminus of Syt-II (residues 8–61) by overlapping PCR, and subcloned into pET-28a vector at Nhe / Xho I site. The following additional residues from pET28 vectors were also expressed in the fusion protein: N-terminus before BoNT/B-H C : MGSSHHHHHHSSGLVPRGSHMASM; C-terminus after Syt-II: VLEHHHHHH. Peptide corresponding to the toxin-binding site in rat Syt-II (residues 40–60) was synthesized (>95% purity) by JPT Peptide Technologies Gmbh (Germany). Protein expression and purification Double His-6 tagged BoNT/B-H C – Syt-II was expressed in E. coli (BL21 strain). The cells were grown in terrific broth medium containing 50 μg ml −1 kanamycin, and grown in 2 l flasks at 37 °C, pH 7.0, with addition of air to mix the medium and maintain an excess of oxygen, to an OD 600 of ~1.5. The temperature was then lowered to 20 °C, and expression induced by the addition of IPTG with a final concentration of 1 mM. After overnight induction, the cells were harvested and frozen in −80 °C. For protein purification, the pelleted cells were thawed, resuspended to an OD600 of ~100 in 50 mM KPi, pH 7.5, 300 mM NaCl and 10% glycerol. Lysation was performed by passing the cell suspension two times through an Emulsiflex-C3 (Avestin, Germany) at 20 kPsi. Unlysed cells and cell debri was spun down via ultra-centrifugation at 4 °C, 267,000 g for 60 min. The supernatant was collected, imidazole, pH 7.8, was added to a final concentration of 12 mM, and incubated with 0.5 ml Ni-NTA per 10 ml supernatant at 4 °C for 60 min, rotating. The material was then packed in a disposable 10 ml column (BioRad), washed 20 column volumes with wash buffer (50 mM HEPES, pH 7.8, 300 mM NaCl and 45 mM imidazole, pH 7.8). The protein was then eluted using wash buffer supplemented with 500 mM imidazole, pH 7.8. Purification was then finished by running the protein over a Superdex 200 10/300GL size exclusion column, pre-equilibrated with 20 mM HEPES, pH 7.0 and 150 mM NaCl. The peak fractions were pooled and concentrated to 5.0 mg ml −1 , using a 30-kDa molecular weight cutoff spin concentrator (Vivaspin). Glycerol was then added to a final concentration of 10%, and the protein was subsequently flash frozen in liquid nitrogen and stored at −80 °C. Expression and purification of BoNT/B-E C for ITC experiments was performed in the same way as BoNT/B-H C – SytII, with the exception that BoNT/B-H C was not frozen, and the final buffer in the size exclusion chromatography was 20 mM KPi, pH 7.0, 150 mM NaCl. Crystallization and structure determination Purified protein was thawed, GD1a oligosaccharide (Elicityl, France) was added to a final concentration of 2.5 mM, and was subsequently crystallized using the vapour diffusion technique. Diffraction quality crystals grew from a solution containing 0.2 M MgCl 2 , 0.1 M HEPES pH 7.0–7.2 and 20–24% PEG 6000. Crystals appeared between 8 and 12 weeks. For cryo protection, they were washed in mother liquor supplemented with 40% PEG 6000, and subsequently flash frozen in liquid nitrogen. Diffraction data was collected at 0.918 Å at beamline 14.1, BESSY, Berlin. The crystals diffracted to 2.3 Å, and were in space group P2 1 . Data processing and reduction were carried out using XDS [39] and programs from the CCP4 suite [40] . Relevant statistics are shown in Table 1 . The structure was solved via molecular replacement, using the previously solved structure of BoNT/B as a search model (PDB code: 2NM1 ). A few cycles of refinement in Refmac5 and Phenix.refine [41] , [42] , interspersed with model building using Coot [43] , were needed to build the full model and its ligands. The final structure contains residues 862–1291, with the exception of two loops, 1152–1158 and 1246–1252 that had ambiguous electron density. At the N-terminus, 6 residues of BoNT/B are missing (MNSEIL), as well as the N-terminal tag. The Syt-II-binding domain, residues 45–59, has well-defined electron density, leaving residues 1–44 of Syt-II (which acts as a linker in this construct) flexible. Furthermore, the entire GD1a molecule is visible in the electron density. The highest resolution data, to 2.3 Å, had a twin fraction of ca. 35%, as analyzed via phenix.xtriage [42] . The structure was therefore refined using twin refinement. Another crystal form, in space group C2, diffracted to 2.6 Å and did not have twinning. The structure was also solved with this data, which was not twinned, and used for comparison with the higher resolution structure obtained from the twinned data. Final R work / R free of the untwinned data was 21.5/26.1%. No substantial differences were observed between the two structures, and as the twinned data with higher resolution gave better final electron density, we choose to use that data for the final model building. Isothermal titration calorimetry Binding of Syt to BoNT/B-H C was measured via ITC on a ITC200 (GE Healthcare) at 25 °C and 1,000 r.p.m. A volume of 200 μl of BoNT/B-H C (typically concentrated to 10–25 μM, in 20 mM KPi pH 7.5, 150 mM NaCl) was added to the cell. In the case of GD1a oligosaccharide addition, 0.25 mM was added to the protein and incubated for 10 min on ice before adding the protein to the cell. Binding was measured upon addition of Syt-II peptide in a stepwise manner, typically 16 injections of 2.6 μl each, at a concentration of 10–15 times the protein concentration in the cell. The first titration was 0.5 μl, and was subsequently deleted in the data analysis. The analysis was performed using the software provided by the manufacturer. Accession codes: Atomic coordinates and structure factors have been deposited in the Protein Data Bank under accession code 4KBB . How to cite this article: Berntsson, R.P.-A. et al. Structure of dual receptor binding to botulinum neurotoxin B. Nat. Commun. 4:2058 doi: 10.1038/ncomms3058 (2013).